Interfacial mobility scale determines the scale of collective motion and relaxation rate in polymer films Thin polymer films are ubiquitous in manufacturing and medical applications, and there has been intense interest in how film thickness and substrate interactions influence film dynamics. It is appreciated that a polymer–air interfacial layer with enhanced mobility plays an important role in the observed changes and recent studies suggest that the length scale ξ of this interfacial layer is related to film relaxation. In the context of the Adam–Gibbs and random first-order transition models of glass formation, these results provide indirect evidence for a relation between ξ and the scale of collective molecular motion. Here we report direct evidence for a proportionality between ξ and the average length L of string-like particle displacements in simulations of polymer films supported on substrates with variable interaction strength and rigidity. This relation explicitly links ξ to the theoretical scale of cooperatively rearranging regions, offering a promising route to experimentally determine this scale of cooperative motion. Thin polymer films are used for a broad range of applications. However, both the mechanical and dynamical properties of these films change considerably in relation to bulk materials for film thickness approaching the nanoscale. As mechanical and dynamical properties are central for many technological applications, studies of property changes in thin polymer films have focused on changes in molecular mobility, commonly quantified by the glass transition temperature T g [1] , [2] . The observed changes in T g of polymer films are usually interpreted in terms of the local mobility changes near their interfaces. Many studies have reported that a repulsive or neutral wall (such as a free surface) decreases T g [3] , [4] , [5] , [6] , while an attractive substrate typically increases T g [1] , [4] , [7] , [8] , [9] , [10] , [11] , [12] , [13] , [14] , [15] , [16] . However, an attractive smooth surface with a modest interaction strength may also enhance the dynamics [7] , [9] , [10] , [17] , [18] , [19] , demonstrating that the strength of polymer–substrate interactions or surface roughness (or surface patterning) can have significant effects. For supported films, the enhancement or slowing down of dynamics induced by two different interfaces complicates the interpretation of the thickness dependence of T g [3] , [4] , [5] , [9] , [11] , [12] , [13] , [14] , [19] . Moreover, some experiments suggest an interfacial scale associated with these dynamical changes [20] , [21] , [22] . For bulk glass formers, the Adam–Gibbs (AG) [23] and random first-order transition (RFOT) [24] theories both argue that there is an intrinsic scale that controls the variation of relaxation approaching T g . Our recent works [25] , [26] , [27] provide evidence that this scale can be related to the characteristic scale of the string-like cooperative motion, providing a molecular realization of the abstract cooperatively rearranging regions (CRRs) invoked by AG and RFOT. However, direct experimental observations of this string-like cooperative motion in molecular glass-forming liquids remains a challenge. Since films exhibit a quantifiable scale for the perturbation of interfacial dynamics [19] , it is natural to ask to what degree this scale relates to the scale of CRR. Stephenson and Wolynes [28] have argued, based on the RFOT theory and scaling arguments, that the interfacial mobility length of films should scale inversely to the configurational entropy of the films. When this result is combined with results showing that the string length scales inversely to the configurational entropy [26] , then we might expect the interfacial mobility length to scale in proportion to the average string length L , and thus describe the temperature T dependence of relaxation. Very recently, Lang and Simmons [29] indeed found that the interfacial mobility scale grows in proportion to the apparent activation energy for relaxation in molecular dynamics simulations of polymer films, suggesting that this scale might provide an estimate of the collective motion scale from the AG model. Our previous study [26] also showed that RFOT is consistent with our observations of string-like collective motion if the size of the ‘entropic droplets’ of this model is equated to the radius of gyration of the strings, further motivating the investigation of the potential direct relation between the scale of string-like collective motion and the interfacial mobility scale. In this study, we address how the dynamics of polymer films supported on rough or smooth surfaces with variable substrate interaction strength can be related with the average string size L , and indeed find that L varies linearly with the scale of the mobility gradient at the polymer–air interface to a good approximation. This offers a promising route to experimentally probe the scale of cooperative relaxation. Dependence of the film dynamics on substrate As a baseline to understand the changes of interfacial scales and cooperative dynamics in films, we need to know the changes in the overall relaxation dynamics as we vary film thickness and substrate properties. Such changes have been considered in previous works [5] , [7] , [19] , [30] , [31] , [32] , where it has been shown that T g for a smooth substrate is typically reduced, while T g for a rough substrate increases. To provide a reference for the dynamical behaviour of our films, we evaluate the mean dynamics as measured by the coherent intermediate scattering function [33] . Relative to the bulk system, the relaxation time of polymer films on the smooth surface decreases as we decrease film thickness ( Fig. 1a ), and these deviations become more pronounced as we decrease T , consistent with our previous studies [19] . As expected, we find an opposite behaviour for the rough surface. We find that changes more rapidly with T for thinner films, that is, a more ‘fragile’ behaviour, resulting in a larger relaxation time relative to the bulk system ( Fig. 1b ). 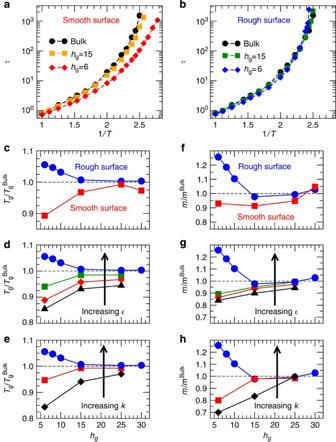Figure 1: Changes of film dynamics due to confinement and substrate interaction. TheTdependence of relaxation timeof a bulk system and two representative film thicknesses supported on a (a) smooth or (b) rough surface. In thisTrange, it is apparent that relative to the bulk,decreases as we decrease the thickness for the film supported on a smooth substrate; in contrast, films supported on a rough substrate show the opposite behaviour. Changes indetermine the changes to the glass transition temperatureTgand fragilitym. (c)Tgrelative to the bulk as a function of film thickness.Tgof films supported on the rough surface increases, while the opposite occurs for a smooth substrate. (d) For the rough substrate,Tgincreases with increasing substrate attraction and (e) increasing surface rigidity. The interaction strengths indare (from bottom to top)εmw=0.477, 0.6, 0.8 and 1.0. The surface rigidity parameters ineare (from bottom to top)k=10, 50 and 100. The topTgcurve inc,dandeis for the sameε=1.0 andk=100, corresponding to thedata inb. Panelsf–hshow the fragilitymfor the same systems shown in panelsc–e. We estimate T g by fitting our data using the Vogel-Fulcher-Tammann (VFT) equation Figure 1: Changes of film dynamics due to confinement and substrate interaction. The T dependence of relaxation time of a bulk system and two representative film thicknesses supported on a ( a ) smooth or ( b ) rough surface. In this T range, it is apparent that relative to the bulk, decreases as we decrease the thickness for the film supported on a smooth substrate; in contrast, films supported on a rough substrate show the opposite behaviour. Changes in determine the changes to the glass transition temperature T g and fragility m . ( c ) T g relative to the bulk as a function of film thickness. T g of films supported on the rough surface increases, while the opposite occurs for a smooth substrate. ( d ) For the rough substrate, T g increases with increasing substrate attraction and ( e ) increasing surface rigidity. The interaction strengths in d are (from bottom to top) ε mw =0.477, 0.6, 0.8 and 1.0. The surface rigidity parameters in e are (from bottom to top) k =10, 50 and 100. The top T g curve in c , d and e is for the same ε =1.0 and k =100, corresponding to the data in b . Panels f – h show the fragility m for the same systems shown in panels c – e . Full size image More specifically, we define T g as the temperature where the extrapolated is a factor of 10 15 times larger than its high T vibrational value (on the order of 10 −13 s), corresponding to the common experimental definition . This definition is not unique, and T g is also frequently defined by the loss of equilibrium at a fixed cooling/heating rate. In the case of experiments, the values obtained for T g by these two approaches are nearly identical, as heating and cooling rates are commensurate with the rough 100 s criterion. In the case of simulations, the T g values from these two methods are dramatically different, simply because the accessible cooling rates for simulation are much faster (by a factor of as much as 10 8 ) than those of experiments. Given the possible confusion that can arrise from a definition that probes a drastically different time scale than experiments, we report the value from the ‘100 s rule’, which conforms better with experimentally defined T g values. Figure 1c shows that, relative to the bulk, T g of polymer films on a rough surface increases with decreasing film thickness, while for the smooth surfaces T g decreases with decreasing film thickness. This is consistent with many previous studies [5] , [7] , [19] , [30] , [31] , [32] . For the rough substrate, we also study a variety of substrate interaction strengths and substrate rigidities. This allows us to tune the T g changes, as decreasing substrate interaction or rigidity decreases T g ( Fig. 1d,e ). Along with T g changes, we expect changes to the fragility, m , which quantifies the T dependence of relaxation near T g . Formally, m is defined as the logarithmic slope of near T g , We evaluate m from the same fit used to estimate T g . Experimentally, m is often found to vary in proportion to T g [34] . Figure 1f–h show a correlation between T g and m for all films, but this relation is not strictly proportional, expected from recent studies [19] , [35] . The slowing down of dynamics approaching the glass transition is characterized by several characteristic transition temperatures, in addition to T g . For the present discussion, the next most relevant temperature is the ‘onset’ temperature for complex liquid dynamics on cooling. At T well above T g , the onset temperature can be defined by the temperature T A where relaxation departs from simple Arrhenius behavour (typically, ). As Fig. 2a shows, the crossover from Arrhenius to non-Arrhenius relaxation occurs in a smooth fashion, making T A difficult to define precisely. Nonetheless, it is apparent that T A ≈0.6 and that T A does not change significantly for different thicknesses or substrate properties. 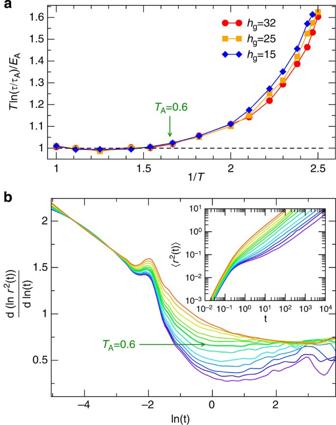Figure 2: Estimation of the onset temperatureTAfor complex dynamics. (a) Rescaled Arrhenius plot of the relaxation time. The symbols represent the simulated data and the dashed line illustrates its high temperature Arrhenius behaviour. AboveT≈0.6,conforms to Arrhenius behaviour. (b) Estimation ofTAusing the logarithmic derivative of the mean-square displacement (equation (7)). For T≳0.6, ∂ ln ‹r2(t)›/∂ lnthas no local minimum near 1 ps. The inset illustrates the time dependence of ‹r2(t)›. The colour gradient of the lines represents the range of temperatures simulated. Figure 2: Estimation of the onset temperature T A for complex dynamics. ( a ) Rescaled Arrhenius plot of the relaxation time . The symbols represent the simulated data and the dashed line illustrates its high temperature Arrhenius behaviour. Above T ≈0.6, conforms to Arrhenius behaviour. ( b ) Estimation of T A using the logarithmic derivative of the mean-square displacement (equation (7)). For T ≳ 0.6, ∂ ln ‹ r 2 ( t )›/∂ ln t has no local minimum near 1 ps. The inset illustrates the time dependence of ‹ r 2 ( t )›. The colour gradient of the lines represents the range of temperatures simulated. Full size image As a consistency check, we also consider that coincident with non-Arrhenius T dependence, single-particle motion becomes caged due to the transient trapping by neighbouring particles. This caging is characterized by the emergence of a plateau in the mean-square displacement ‹ r 2 ( t )› around T A . Therefore, as an alternate method to estimate of T A , we identify the lowest temperature at which the logarithmic derivative, has no local minimum near 1 ps, the characteristic scale for particle caging. Figure 2b shows the logarithmic derivative for a representative film, which indicates the vanishing of a plateau at T A ≈0.6, consistent with our estimate from . Relation between interfacial and cooperative motion The changes of T g are due in part to the enhancement or suppression of dynamics in the interfacial regions, as qualitatively illustrated in Fig. 3 . It is precisely the scale of this interfacial region on which we now focus our attention. To quantify interfacial dynamics and the corresponding interfacial length scale, we resolve the dynamics locally. We first contrast the local dynamics as function of distance z from the substrate boundary of the rough or smooth surfaces with ε mw =1. To do so, we evaluate the self-part of the dynamical density correlation function [33] and condition it by the the distance z from the substrate in intervals δz =0.875. From this, we obtain the distance-dependent self relaxation time . Figure 4a shows that starting from the free interface (large z ), to the film centre, has nearly the same z dependence for rough or smooth surfaces; differs for rough and smooth substrate at distances close to the surface ( z =0). 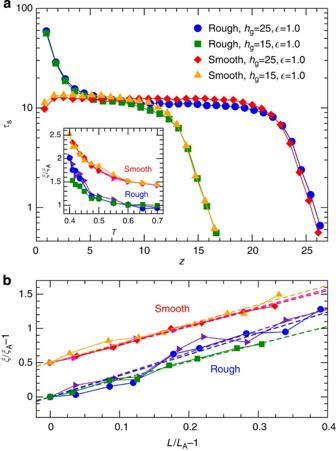Figure 4: Interfacial scale of films with smooth or rough substrates. (a) The local relaxation timeas function of distancezfrom the substrate for films supported on a rough or smooth surface. The inset shows the resulting free surface mobile layer scale,ξ, for films supported on a rough or smooth substrate as function of temperatureT;ξis normalized by its value atTA. We also showξdata for thickness 32 (triangle right) in the inset. The values ofξfor the smooth surface are shifted by 0.5 for clarity. (b)ξ/ξA−1 for films supported on a rough or smooth surface as a function ofL/LA−1, showing proportionality between these quantities. The dashed lines indicate a linear proportionality. The normalizedξ/ξA−1 values of films on a smooth surface are shifted by 0.5 for clarity of the figure. Specifically, increases close to the rough surface but decreases near the smooth surface. Similar results occur for rough substrates with variable interaction strength and rigidity ( Fig. 5 ), as discussed below. The enhanced dynamics near the smooth surface is a consequence of the fact the monomers can ‘slide’ along the substrate due its smoothness; hence, that relaxation parallel to the substrate is more rapid than relaxation perpendicular to the substrate (see refs 19 , 32 ). 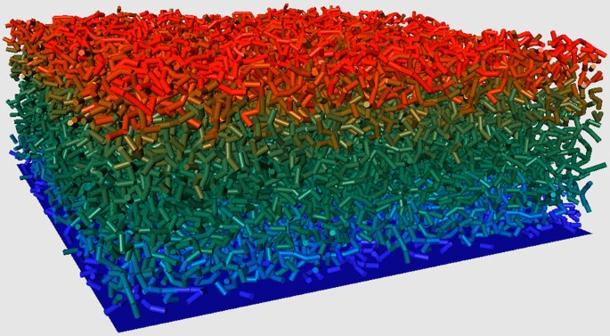This anisotropy disappears for the rough surface that we study. Figure 3: Visualization of the polymer film relaxation gradient. The tubes represent the segments of the simulated polymer film of thicknesshg=15, supported on a rough substrate. The colour gradient describes the local relaxation time as a function of distance from the substrate (seeFig. 4): the slowest relaxing chains are coloured blue, while the most rapidly relaxing chains are shown in red. This illustration makes visually apparent the existence of a substrate, central and free-surface region of the film. Figure 3: Visualization of the polymer film relaxation gradient. The tubes represent the segments of the simulated polymer film of thickness h g =15, supported on a rough substrate. The colour gradient describes the local relaxation time as a function of distance from the substrate (see Fig. 4 ): the slowest relaxing chains are coloured blue, while the most rapidly relaxing chains are shown in red. This illustration makes visually apparent the existence of a substrate, central and free-surface region of the film. Full size image Figure 4: Interfacial scale of films with smooth or rough substrates. ( a ) The local relaxation time as function of distance z from the substrate for films supported on a rough or smooth surface. The inset shows the resulting free surface mobile layer scale, ξ , for films supported on a rough or smooth substrate as function of temperature T ; ξ is normalized by its value at T A . We also show ξ data for thickness 32 (triangle right) in the inset. The values of ξ for the smooth surface are shifted by 0.5 for clarity. ( b ) ξ / ξ A −1 for films supported on a rough or smooth surface as a function of L / L A −1, showing proportionality between these quantities. The dashed lines indicate a linear proportionality. The normalized ξ / ξ A −1 values of films on a smooth surface are shifted by 0.5 for clarity of the figure. 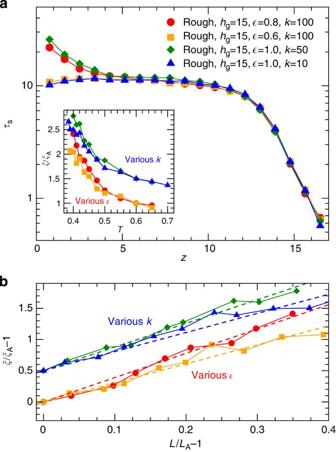Figure 5: Interfacial scale of films with a rough substrate of variable attraction and flexibility. (a) The local relaxation timeas function of distancezfrom the substrate for various interfacial energiesεwmand surface rigiditiesk. The inset shows mobile layer scalesξfor films supported on a rough surface with variousεandkas function of temperatureT, whereξis normalized by its value atTA. The values ofξfor substrate with differentkare shifted by 0.5 for clarity. (b)ξ/ξA−1 for films supported on rough surface as function ofL/LA−1, indicating their apparent proportionality. The dashed lines indicate a linear proportionality. The normalizedξ/ξA−1 values for substrates with differentkare shifted by 0.5 for clarity of the figure. Full size image Figure 5: Interfacial scale of films with a rough substrate of variable attraction and flexibility. ( a ) The local relaxation time as function of distance z from the substrate for various interfacial energies ε wm and surface rigidities k . The inset shows mobile layer scales ξ for films supported on a rough surface with various ε and k as function of temperature T , where ξ is normalized by its value at T A . The values of ξ for substrate with different k are shifted by 0.5 for clarity. ( b ) ξ / ξ A −1 for films supported on rough surface as function of L / L A −1, indicating their apparent proportionality. The dashed lines indicate a linear proportionality. The normalized ξ / ξ A −1 values for substrates with different k are shifted by 0.5 for clarity of the figure. Full size image We next quantify the dynamical length scale ξ of the free-interface (mobile-layer scale) based on local relaxation time near the free surface, as we did in our previous work (see ref. 19 for a complete description). A similar choice was examined by Lang and Simmons [29] . We define ξ as the length where deviates by 30% from the nearly constant value at the film centre. The precise condition for the fractional deviation does not affect our qualitative results, provided that the choice is large enough that fluctuations in do not play a role ( ≳ 15% for these data) and small enough to be meaningful ( ≲ 50%). 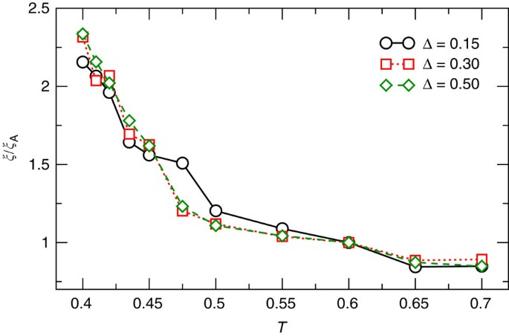Figure 6: Sensitivity of the interfacial scale to its definition. Interfacial mobility scaleξdefined by the length wheredeviates by 15%, 30% or 50% from the nearly constant value at the film centre. TheTdependence for all choices is nearly identical. The values ofξare normalized by their values atTAto remove the trivial effect of changing the cutoff percentage. Figure 6 demonstrates the robustness of our definition of ξ for several cutoff choices. It is apparent that the choice of the cutoff does not change our qualitative findings. Figure 6: Sensitivity of the interfacial scale to its definition. Interfacial mobility scale ξ defined by the length where deviates by 15%, 30% or 50% from the nearly constant value at the film centre. The T dependence for all choices is nearly identical. The values of ξ are normalized by their values at T A to remove the trivial effect of changing the cutoff percentage. Full size image An advantage of this definition for the interfacial scale is that it depends both on the behaviour near the interface, as well as the film interior. We find below that both contributions are important for our results. Note that the bulk material does not provide a useful reference to define ξ , as the dynamics near the centre of the film often differs from the bulk [19] . We limit our analysis to films in which the interfacial scale is no larger than half of the film thickness [19] . The inset of Fig. 4a shows the growth of ξ with decreasing T for four representative films supported on a rough or smooth surface. The growth of this dynamical length scales has been observed in previous studies, where the scale is inferred in a similar fashion [17] , [19] , [29] , [36] . We emphasize that this interfacial mobility scale is distinct from the scale of interfacial density changes; hence, there is no simple relation between mobility and local density [19] . Note that ξ is normalized by its value ξ A at the onset temperature T A for ‘slow’ dynamics. For our films T A ≈0.6, (see Fig. 2 ). We next consider the possible relation of the interfacial scale to a dynamical heterogeneity scale. Glass-forming liquids generally exhibit dynamical heterogeneity, typically manifested by spatial correlations of particle mobility. In particular, those monomers with the greatest mobility tend to cluster and subsets within these clusters move collectively in a string-like manner, observed both in computer simulations [23] , [26] , [37] , [38] , [39] , [40] , [41] , [42] , [43] and colloidal experiments [44] , [45] , [46] , [47] . Significantly, several publications [25] , [26] , [27] , [48] indicate that the string size may offer a molecular realization of CRR. Therefore, we aim to test whether the interfacial scale might be reflective of this scale of cooperative motion. Accordingly, we need to evaluate the average size of string-like cooperative motion, L ( T ). We evaluate L ( T ) following the methods described in ref. 26 . Figure 4b shows that L and ξ grow proportionally, relative to their values ξ A and L A at the onset temperature T A , where the proportionality constant A fluctuates with no apparent trend around a mean A =0.32. For reference, the values of L ( T A ) and ξ ( T A ) are relatively constant for all systems; specifically, L A ≈1.41 and ξ A ≈3.6. Moreover, the precise values used for ξ A and L A are not critical for our findings. Given that L varies inversely proportional to the configurational entropy S conf [26] , ξ should also vary inversely proportional to S conf (with the factors of ξ A and L A included). Indeed, Stephenson and Wolynes [28] predict a direct inverse proportionality, but our findings show this relation must include an additive term accounting for the scales of collective motion at T A . This provides our first indication that the interfacial scale might indeed reflect a fundamental heterogeneity scale. To further test of the robustness of this relation between interfacial and heterogeneity scales, we extend our analysis to consider variations in surface–polymer interaction strength ε wm and surface rigidity k . Analogous to shown for smooth and rough surfaces, Fig. 5a , shows increases near the substrate as we increase ε wm , since stronger interfacial interactions enhance the trapping of monomers near the attractive substrate. Likewise, decreasing wall rigidity k allows monomers to move more freely, as the wall atoms are less strongly localized. From these data we obtain ξ , as done for the previous case. The dependence of ξ on ε wm and k is not obvious, as appears nearly identical near the free surface for various ε wm and k . However, the behaviour near the interface and at the film centre play a role in determining the variation of ξ . As the values for near the film centre vary with both ε wm and k , we find a modest, but non-trivial difference in ξ as the suface properties change. Figure 5a inset shows that ξ increases on cooling (similar to Fig. 4a , inset). Moreover, Fig. 5b confirms the apparent proportional variation between in ξ / ξ A −1 and L / L A −1, consistent with our findings in Fig. 4b . This supports the hypothesis that ξ and L are related. Connection to film relaxation To demonstrate the practical and physical importance of such a relation, we now consider how ξ may be related to , and hence T g . Central to both the AG and RFOT descriptions of glass formation is the idea that the activation free energy for relaxation grows with the cooperativity scale. In recent works [25] , [26] , [27] , we have offered computational evidence that L provides a measure of the extent of collective motion (that is, the CRR) consistent with the ideas of both AG and RFOT. Based on this ‘string model’ for glass formation [49] , (for the entire film) is related to the average string size L by where Δ μ is the limiting activation free energy as T → T A . At high temperatures ( T > T A ), has an Arrhenius dependence, and Eyring transition state theory provides a reasonable description of the fluid dynamics. Δ μ contains both enthalpic Δ H and entropic Δ S terms, so that Δ μ =Δ H − T Δ S . 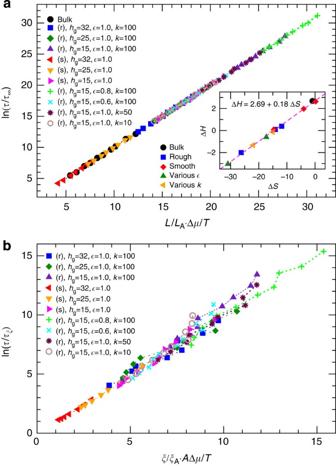Figure 7: Test of the AG relation using string sizeLand interfacial scaleξ. (a) Collapse ofversusL/LA· Δμ/Tfor all systems. (b) Collapse ofversusξ/ξA⋅AΔμ/Tfor all systems. Inset (a) shows the proportionality between ΔHversus ΔSfor all systems with an entropy–enthalpy compensation temperature slopeTcomp≈0.2. Figure 7a confirms the applicability of the string size to quantify dynamical changes in polymer films under all conditions examined, including variable film thickness, surface roughness and polymer–substrate interaction. Although such a relation has been shown in bulk and polymer composite systems [25] , [26] , [27] , here we demonstrate the applicability to polymer films for a wide range of surface conditions and film thicknesses. The remarkable degree of data collapse in Fig. 7a provides strong evidence supporting the identification of the strings with the abstract CRR of AG. Figure 7: Test of the AG relation using string size L and interfacial scale ξ . ( a ) Collapse of versus L / L A · Δμ/ T for all systems. ( b ) Collapse of versus ξ / ξ A ⋅ A Δμ/ T for all systems. Inset ( a ) shows the proportionality between Δ H versus Δ S for all systems with an entropy–enthalpy compensation temperature slope T comp ≈0.2. Full size image As there is no readily accessible experimental measurement of string-like cooperative motions, and as we found an apparent proportionality between L and the interfacial scale ξ , we consider if ξ can be used as a substitute for L . Combining equations (4) and (5) suggests an AG-like relation between and ξ , Our data indicate that the T dependence of the leading term exp[(1− A )Δμ/ k B T ] is weak in comparison with the term involving ξ , both because 1− A is relatively small and as ξ grows on cooling. Consequently, if one approximates the first exponential term as constant, the expression simplifies to more generally, without approximation . The approximation that is constant and is important for possible experimental application, as L (and hence A ) is not easily measured. Using this approximation, we find that ξ works nearly as well as L to describe using the same Δ H and Δ S values already determined from the relation of with L . In other words, we do not allow these parameters to be refit. This parameterization results a collapse of all data shown in Fig. 7b . This provides direct evidence that the interfacial dynamical scale contains the information on changes to CRR size that are fundamental to the AG and RFOT approaches. The data collapse shown in Fig. 7 depends on the parameters Δ H and Δ S . Thus, it is natural to consider how these quantities vary. Curiously, the inset of Fig. 7a shows a linear dependence between Δ H and Δ S , the slope of which defines an entropy–enthalpy ‘compensation temperature’ T comp ≈0.2. The origin of this particular value poses an interesting question for future study. The high interfacial mobility of both glassy and crystalline materials is a problem of profound importance for both a fundamental understanding of glass formation and technological applications. The physical picture, derived from both the classical AG theory and the more recent RFOT theory, suggests that the strong temperature dependence of relaxation times in glass-forming liquids derives from the growing extent of the collective motion on cooling, and our findings support interpreting the string size as this scale of collective motion. We further address how the dynamical interfacial layer might be related to collective molecular motion. Stephen and Wolynes [28] argued, from a purely theoretical standpoint, that the interfacial mobility scale is inversely proportional to the configurational entropy S conf [26] , which implies that the interfacial scale ξ of glass-forming liquids should scale in direct proportionality to the CRR scale of AG theory. We have shown the validity of an AG-like relation of L to and to ξ for a variety of surface energies and for a range of boundary stiffnesses on model rough and smooth surfaces, and expect these relations to be very useful in applications. Lang and Simmons [29] recently observed a relation between and ξ mathematically equivalent to equation (7) where, in effect, the constants and A in the prefactor and exponent were freely adjusted to fit their relaxation time data for a similar coarse-grained polymer model. They did not quantify collective motion in their films; hence, their findings were only suggestive of a relation between ξ and the CRR scale. We point out that our relation between , L and ξ does not account for the varying relaxation time (and corresponding mobility variation) across the film profile. However, there is a basic rationale for choosing this approach. From the underlying theory, dynamical changes are rooted in variation of the configurational entropy S conf , which can only be defined for the system as a whole. Accordingly, the application of AG-like ideas is more appropriate for relaxation and cooperative motion within the film as a whole. Of course, as strings consist of highly mobile particles, and as these particles are more numerous near the free interface [40] , the average L we evaluate is strongly influenced by the interfacial collective motion. This may be an important underlying factor for the apparent relation between the interfacial scale ξ and L . Interestingly, the length of the strings tends to be shorter in the interfacial region, perhaps explaining the near-Arrhenius relaxation observed in the interfacial dynamics [19] , but the investigation of this phenomenon will require further study. Our findings help to advance our understanding of collective motion in glassy materials and the impact of these collective motions on the interfacial mobility of glassy materials. At the same time, our results suggest a practical metrology for estimating changes in the scale of collective motion in glassy materials that might be used in the design of advanced materials. An important aspect of our work is that it opens a possible route to indirectly access the cooperativity scale in experiments. A similar relation between the scale of cooperative motion, the interfacial mobility scale and the ‘coloured noise’ exponent describing particle displacement fluctuations was found in the glassy interfacial zone of Ni nanoparticles [50] , [51] ; however, this suggested relation has not been confirmed in ordinary glass-forming liquids. Tanaka and coworkers [52] have also found a relationship between the interfacial mobility scale as we have defined it and a correlation length associated with clusters having high local order and a class of particles that is highly immobile. The observations of the present work suggests that there might be complementarity between these different types of clusters of extreme mobility, and future work should explore this relationship quantitatively. Simulation model Our findings are based on equilibrium molecular dynamics simulations of a coarse-grained representation of polymer chains supported on a substrate with variable surface rigidity and interaction strength. Specifically, we consider (i) a perfectly smooth substrate and (ii) an atomistically rough surface, where the surface rigidity is controlled by the lattice binding strength. Non-bonded monomers and rough wall atoms interact with each other via a Lennard–Jones (LJ) potential, where a ‘force-shifted’ truncation is used at r c =2.5 σ ij (ref. 53 ). The index pair ij distinguishes monomer–monomer (mm), wall–monomer (wm) and wall–wall (ww) interactions. The LJ interaction is not included for the nearest bonded neighbours along the chain. Bonded monomers are connected by a harmonic spring potential U bond = κ /2 ( r − r 0 ) 2 with bond length r 0 =0.9 σ mm to avoid crystallization, and a spring constant κ =(1111) ε mm /σ mm 2 (ref. 17 ). We use this harmonic bond potential, rather than the often used ‘FENE’ bond potential [54] , due to crystallization that we find using the FENE potential for films on rough surfaces. Reference [55] 55 has considered a more detailed study of this phenomenon. For the perfectly smooth substrate, the interaction between a monomer and the substrate is given by a ‘9–3’ LJ potential, where z is the distance of a monomer from the wall and ρ wall is the number density of wall sites. This is the same model that we studied in recent work [19] . To model the rough wall, we follow the model described by refs 16 , 56 . Specifically we tether a single layer of wall atoms to the sites of triangular lattice ((111) face of an FCC lattice) with a harmonic potential , where denotes the equilibrium position of atom i within the triangular lattice and k is the harmonic spring constant [16] , [56] . We choose the interaction strength between wall particles ε ww =1.0, and equilibrium distance between nearest neighbours to be 2 1/6 σ ww , where σ ww =0.80 σ mm (which also sets ρ wall for the smooth surface). Note that we have slightly changed the bead size σ ww from the previous work [16] , [56] to suppress crystallization of the film. An additional smooth wall is placed behind the explicit layer to make sure that polymers do not penetrate the walls. We use various substrate interaction strengths ε wm between the rough surface and polymers, ranging from 0.4 to 1.0 ε mm (with a fixed k =100); we vary the rigidity of the wall by changing k from 10 to 100 (with a fixed ε wm =1). To study the dynamical changes in polymer films, we simulate systems with a number of chains N c =200, 300, 400, 600, 1,000, or 1,200 chains of 10 monomers with lateral dimensions L x ≈20 σ and L y ≈20 σ . These sizes correspond to thicknesses from ≈6–32 monomer diameters. In addition, we simulate a pure bulk system at zero pressure that consists of 400 chains of 10 monomers each. All values are in reduced units where σ mm =1 and ε mm =1, temperature in units of ε / k B ( k B is Boltzmann’s constant) and time in unit of ( mσ mm 2 / ε mm ) 1/2 . In physical units relevant to real polymer materials, ε ≈1 kJ mol −1 for a polymer (similar to polystyrene) with T g ≈100 °C, and the length of a chain segments σ is typically ≈1–2 nm. Molecular dynamics calculations Simulations were carried out using ‘in-house’ code written and developed since the mid 1990, s. The equations of motion are integrated via the reversible reference system propagator algorithm, a multiple time-step algorithm [57] . We use a velocity Verlet version of reversible reference system propagator algorithm with the forces separated into bonded (fast) and non-bonded (slow) components. For each update of the non-bonded forces, there are three updates of the bond forces with an integration step of 0.002. The temperature is controlled using the Nose–Hoover method [53] . We select the ‘mass’ of the thermostat Q =6 NT / ω 2 where ω =234.09 is the intrinsic frequency for a face-centred cubic LJ system [58] , a natural frequency for the heat bath. The systems are prepared by first equilibrating a film confined between two surfaces at relatively high T =1.0 for at least 2,000 LJ time units (10 6 integration steps). The upper surface is then removed to create a supported film, which is cooled to the desired temperature. We carry out preliminary runs at each T to estimate the relaxation time of the coherent intermediate scattering function at the wave vector of the first peak in the structure factor, where is slowest (excepting the limiting case q → 0). Based on this, we ensure that equilibration runs are at least 10 times in length, and production runs (from which data are analysed) are a further 10–100 time in length. We further check for any systematic aging in production runs by evaluating correlation functions for multiple waiting times. Any production runs that do not satisfy these criteria are either re-run for longer times to satisfy the criteria, or eliminated if run times become prohibitive. At the lowest T studied, equilibration typically extends over a minimum of 50 × 10 3 LJ time units. How to cite this article: Hanakata, P. Z. et al. Interfacial mobility scale determines the scale of collective motion and relaxation rate in polymer films. Nat. Commun. 5:4163 doi: 10.1038/ncomms5163 (2014).